High rates of photobiological H2production by a cyanobacterium under aerobic conditions Among the emerging renewable and green energy sources, biohydrogen stands out as an appealing choice. Hydrogen can be produced by certain groups of microorganisms that possess functional nitrogenase and/or bidirectional hydrogenases. In particular, the potential of photobiological hydrogen production by oxygenic photosynthetic microbes has attracted significant interest. However, nitrogenase and hydrogenase are generally oxygen sensitive, and require protective mechanisms to function in an aerobic extracellular environment. Here, we describe Cyanothece sp. ATCC 51142, a unicellular, diazotrophic cyanobacterium with the capacity to generate high levels of hydrogen under aerobic conditions. Wild-type Cyanothece 51142 can produce hydrogen at rates as high as 465 μmol per mg of chlorophyll per hour in the presence of glycerol. Hydrogen production in this strain is mediated by an efficient nitrogenase system, which can be manipulated to convert solar energy into hydrogen at rates that are several fold higher, compared with any previously described wild-type hydrogen-producing photosynthetic microbe. Microbial H 2 production relies on either photosynthetic or fermentative processes. Economic feasibility studies suggest that a direct and efficient conversion of solar energy to H 2 in a carbon-neutral way is necessary for the process to be commercially viable [1] , [2] . Several photosynthetic microalgal and bacterial species possessing nitrogenase and/or hydrogenase enzymes are being studied as prospective model organisms for photobiological H 2 production [3] , [4] , [5] . Outstanding among them are Rhodopseudomonas palustris , a purple photosynthetic, nitrogen-fixing bacterium; Chlamydomonas reinhardtii , a green eukaryotic alga; as well as Anabaena and Synechocystis , members of the cyanobacterial group. High specific rates of nitrogenase-mediated H 2 production have been reported for R. palustris [6] . However, R. palustris performs anoxygenic photosynthesis, thereby requiring an anaerobic environment for photobiological H 2 production [7] , [8] , [9] . Anabaena , a filamentous diazotrophic cyanobacterial strain, produces H 2 in heterocysts, specialized N 2 -fixing cells, which maintain a microaerobic environment to protect the oxygen-sensitive nitrogenase enzyme. However, the low frequency of heterocysts in a filament (about one in ten cells normally differentiates into heterocysts [10] ) consequently results in modest yields of net H 2 production. In contrast, H 2 production in C . reinhardtii and Synechocystis sp. PCC 6803 is mediated by hydrogenase enzymes, and H 2 production can be achieved in both of these organisms only under strictly anaerobic conditions [11] , [12] , [13] . Although these strains have long been used as model organisms to study biohydrogen production, the importance of selecting additional novel and native strains with diverse energy conversion systems that might have evolved as a consequence of specific ecological pressure has often been emphasized [1] , [14] . A recent effort in this direction has identified ten native N 2 -fixing, heterocystous cyanobacterial strains that exhibit higher rates of H 2 production compared with some of the previously studied mutant strains [15] . In the present report, we describe Cyanothece sp. ATCC 51142, a cyanobacterial strain with the ability to produce remarkably high amounts of H 2 under aerobic conditions. Cyanothece strains thrive in marine environments limited in dissolved inorganic bioavailable nitrogenous compounds, and have been recognized for their role in maintaining the marine nitrogen cycle [16] , [17] , [18] . Cyanothece 51142 can derive the majority of its nutritional requirements from sunlight, atmospheric carbon dioxide and nitrogen gases ( Fig. 1 ). During the day, it performs photosynthesis and fixes carbon, which is stored as large reserves of glycogen [19] . At the onset of the dark period, high rates of respiration rapidly create a suboxic intracellular environment. This, in turn, facilitates oxygen-sensitive and energy-intensive processes such as N 2 fixation and H 2 production to occur at night at the expense of the accumulated glycogen. The orchestrated diurnal cycling patterns of the central metabolic processes in this organism have recently been described using a global transcriptomic approach [20] . These unique attributes of Cyanothece 51142, which make it an ideal organism for H 2 production, are possibly the remnants of the metabolic and regulatory processes that aided in the acclimatization of ancient cyanobacteria during their transition from an anaerobic to an aerobic environment. Retention of ancient metabolic traits that originated in the Archaean oceans has been reported in other cyanobacterial strains [21] . 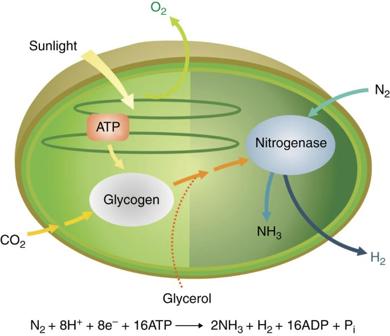Figure 1: Photobiological H2production inCyanothece51142. A schematic diagram showing the process of biohydrogen production byCyanothece51142 cells using solar energy and atmospheric CO2and/or glycerol. CO2is fixed during the day to synthesize glycogen, which serves as an energy reserve and electron source for H2production at night. Figure 1: Photobiological H 2 production in Cyanothece 51142. A schematic diagram showing the process of biohydrogen production by Cyanothece 51142 cells using solar energy and atmospheric CO 2 and/or glycerol. CO 2 is fixed during the day to synthesize glycogen, which serves as an energy reserve and electron source for H 2 production at night. Full size image A two-stage system for photobiological H 2 production We developed a two-stage H 2 production system in Cyanothece 51142 on the basis of our previous knowledge of the diurnal rhythms in this unicellular cyanobacterium [22] , [23] . The two stages were comprised of a growth phase during which cells were allowed to grow aerobically under 12 h light/12 h dark cycles, followed by an incubation phase during which cells sampled at the end of the 12 h light period were incubated in airtight vials under continuous illumination for 12 h. During this latter light-incubation period, the physiological activities of the cells were in step with the subjective dark condition, thereby facilitating N 2 fixation and H 2 production. At the completion of the incubation phase, the headspace of the vials (which contained 100% air at the beginning of incubation) was analysed for H 2 accumulation. We determined that photoautotrophically grown Cyanothece 51142 exhibited high specific rates of H 2 production (>150 μmol of H 2 per mg of chlorophyll per hour (Chl.h) or 2.34 μmol of H 2 per mg of dry weight per hour) under aerobic incubation conditions ( Fig. 2a ). This is striking, as most unicellular photosynthetic microbial strains require a complete anaerobic environment for H 2 production [24] ( Table 1 ). 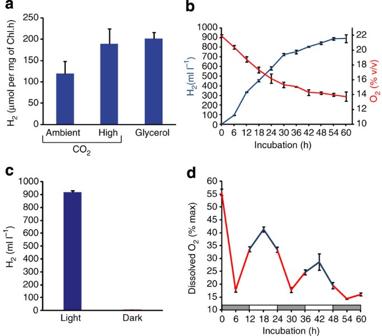Figure 2: Aerobic H2production rates and generation of a suboxic intracellular environment inCyanothece51142. (a) Specific rates of H2production byCyanothece51142 grown under aerobic, photoautotrophic conditions using ambient (0.03%, v/v) or high (8%, v/v) concentrations of CO2, and under photomixotrophic growth conditions with glycerol (50 mM). Cultures were incubated under aerobic conditions for H2production. Each column represents an average of measurements from at least three biological replicates. Error bars indicate s.d. values from the average. (b) Kinetics of aerobic photobiological H2production in a batch culture ofCyanothece51142. H2production (blue) could be observed for more than 60 h in vials containing cultures under aerobic incubation conditions in the presence of light. The respiratory activities of the cells resulted in a gradual decrease in O2concentration in the headspace of the vials (red). Three biological replicates were used for the measurements. Error bars indicate s.d. values from the average. (c) Comparison of cumulative H2accumulation in vials with cells under light and dark incubation conditions. A volume of 916 ml of H2per litre of culture accumulated in the vials when incubated in the light compared with 7 ml of H2per litre of culture accumulation in the dark. Each column represents an average of measurements from at least three biological replicates. Error bars indicate s.d. values from the average. (d) Dissolved O2levels in a batch culture ofCyanothece51142 cells under H2-producing conditions. The circadian rhythms of respiratory and photosynthetic activities were reflected in the dissolved O2concentration of the culture. The culture was transferred to incubation vials at the beginning of the dark period when the dissolved O2level was about 50% of the maximum (assuming 100% equals 230 μM dissolved O2at 30 °C). The O2concentration reduced starting from the middle of the subjective light period (blue line, grey bar), was at its minimum at the middle of the subjective dark period (red line, white bar), after which an increase was observed because of photosynthetic oxygen evolution. The horizontal bars below thexaxis denote subjective day (open) and night (filled) periods. Three independent biological replicates were used for the measurements. Error bars indicate s.d. values from the average. Figure 2: Aerobic H 2 production rates and generation of a suboxic intracellular environment in Cyanothece 51142. ( a ) Specific rates of H 2 production by Cyanothece 51142 grown under aerobic, photoautotrophic conditions using ambient (0.03%, v/v) or high (8%, v/v) concentrations of CO 2 , and under photomixotrophic growth conditions with glycerol (50 mM). Cultures were incubated under aerobic conditions for H 2 production. Each column represents an average of measurements from at least three biological replicates. Error bars indicate s.d. values from the average. ( b ) Kinetics of aerobic photobiological H 2 production in a batch culture of Cyanothece 51142. H 2 production (blue) could be observed for more than 60 h in vials containing cultures under aerobic incubation conditions in the presence of light. The respiratory activities of the cells resulted in a gradual decrease in O 2 concentration in the headspace of the vials (red). Three biological replicates were used for the measurements. Error bars indicate s.d. values from the average. ( c ) Comparison of cumulative H 2 accumulation in vials with cells under light and dark incubation conditions. A volume of 916 ml of H 2 per litre of culture accumulated in the vials when incubated in the light compared with 7 ml of H 2 per litre of culture accumulation in the dark. Each column represents an average of measurements from at least three biological replicates. Error bars indicate s.d. values from the average. ( d ) Dissolved O 2 levels in a batch culture of Cyanothece 51142 cells under H 2 -producing conditions. The circadian rhythms of respiratory and photosynthetic activities were reflected in the dissolved O 2 concentration of the culture. The culture was transferred to incubation vials at the beginning of the dark period when the dissolved O 2 level was about 50% of the maximum (assuming 100% equals 230 μM dissolved O 2 at 30 °C). The O 2 concentration reduced starting from the middle of the subjective light period (blue line, grey bar), was at its minimum at the middle of the subjective dark period (red line, white bar), after which an increase was observed because of photosynthetic oxygen evolution. The horizontal bars below the x axis denote subjective day (open) and night (filled) periods. Three independent biological replicates were used for the measurements. Error bars indicate s.d. values from the average. Full size image Table 1 Specific rates of H 2 production by wild-type strains of Cyanothece 51142 and other model photosynthetic microbes. Full size table The rates of H 2 production in Cyanothece 51142 could be greatly enhanced when cells were grown in the presence of additional carbon sources, as observed in cultures supplemented with high concentrations of CO 2 , or glycerol ( Fig. 2a ). Cells grown under CO 2 -enriched air and incubated under aerobic conditions could produce 230 μmol of H 2 per mg of Chl.h ( Fig. 2a ). In fact, a batch culture of Cyanothece 51142 cells supplemented with 50 mM glycerol could produce more than 900 ml of H 2 per litre of culture over a period of 2 days ( Fig. 2b,c ) when incubated in constant light under aerobic conditions ( Fig. 2b ). Notably, the kinetics of H 2 production under these conditions revealed high rates even early in the incubation phase when the O 2 concentration in the headspace of the vials was equivalent to that in air ( Fig. 2b ), indicating that an intracellular anoxic environment facilitates nitrogenase activity during the subjective dark period. The O 2 level in the headspace diminished with time ( Fig. 2b ), indicating continued respiratory activities in the cells. Moreover, as shown in the next subsection, transcripts of coxA , the gene encoding subunit A of the cytochrome c oxidase enzyme involved in respiration, were also detected under these conditions. This respiration-induced microaerobic environment was also reflected in the dissolved O 2 levels in the culture in the incubation vials ( Fig. 2d ). A rapid decline in the dissolved O 2 concentration was observed at the beginning of the incubation phase, followed by periodic oscillations in O 2 levels, which corresponded to the respiratory and photosynthetic activity of the cells in the subjective dark and light periods, respectively. In comparison with light incubation, incubation under dark conditions reduced the level of H 2 production by more than 100-fold, indicating that H 2 production in this system is driven by light energy, and the high rates observed cannot be achieved by dark fermentation of glycerol alone ( Fig. 2c ). Additional carbon sources lead to higher glycogen content We assessed the influence of external carbon sources on the cellular energy reserves, a critical determinant of nitrogenase activity and H 2 production. The glycogen levels of the cells were compared between pre- (I 0 ) and post-incubation (I 12 ) samples collected from cultures grown under ambient CO 2 (0.03%), under 8% CO 2 -enriched air, and with 50 mM glycerol. Either high CO 2 or glycerol enhanced the glycogen reserves of the cells ( Fig. 3 ). In ambient and high CO 2 -treated cells, the glycogen level diminished at the end of the incubation period, indicating that the endogenous carbon source was being used for H 2 production ( Fig. 2a ). In contrast, cells grown in the presence of glycerol showed higher levels of glycogen at the end of the 12 h-light incubation phase (I 12 ), implying direct utilization of glycerol as a source of ATP and reductants by the nitrogenase enzyme under this photomixotrophic condition. This is supported by the observation that expression of glycogen phosphorylase ( glgP ), a gene involved in glycogen degradation, was also downregulated in glycerol-supplemented cells ( Fig. 4b ). In this context, we have recently shown that Cyanothece 51142 uses glycerol as the sole carbon source when cells are grown under photomixotrophic conditions in the presence of glycerol [25] . 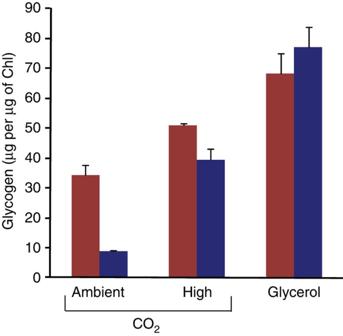Figure 3: Effects of external carbon sources on glycogen accumulation inCyanothece51142. I0(red) and I12(blue) indicate the beginning and end of a 12 h-light incubation period for H2production, respectively. Differences in glycogen level between the two time points correspond to the amount of glycogen used for N2fixation/H2production. Each column represents an average of measurements from at least three biological replicates. Error bars indicate s.d. values from the average. Figure 3: Effects of external carbon sources on glycogen accumulation in Cyanothece 51142. I 0 (red) and I 12 (blue) indicate the beginning and end of a 12 h-light incubation period for H 2 production, respectively. Differences in glycogen level between the two time points correspond to the amount of glycogen used for N 2 fixation/H 2 production. Each column represents an average of measurements from at least three biological replicates. Error bars indicate s.d. values from the average. 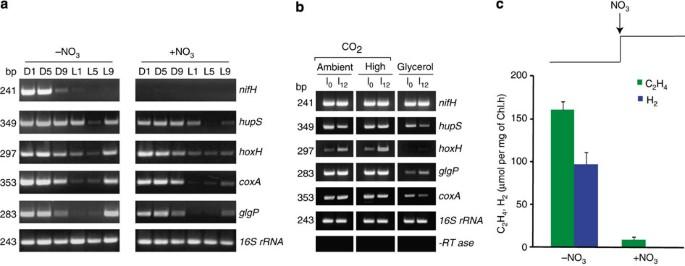Figure 4: H2production inCyanothece51142 is primarily mediated by the nitrogenase enzyme system. (a) Comparisons of the expression of genes involved in H2metabolism under N2-fixing (−NO3) and nitrogen-sufficient (+NO3) conditions from cultures grown under 12 h light/dark cycles.nifHtranscripts could only be observed under N2-fixing condition, whereashoxHandhupStranscripts were present under both conditions.coxAtranscripts were predominant during the dark cycle both under N2-sufficient and N2-deficient conditions. Transcripts forglgPwere abundant during the dark cycle under both conditions. 16SrRNAwas used as the loading control. Cells were collected at 4 h intervals, between D1 (1 h after the onset of the dark cycle) and L9 (9 h into the light cycle). (b) Reverse transcription PCR analysis of the enzyme systems involved in H2metabolism inCyanothece51142. Samples were collected from the incubation bottles (continuous light, aerobic) at the beginning (I0) and end of the incubation phase (I12). StrongnifHexpression could be observed at I0, in the control (grown in ambient CO2) as well as in cultures supplemented with high concentrations of CO2or glycerol.nifHtranscripts were also present in cells incubated under light during H2production (I12). Expression ofglgPwas downregulated in cultures supplemented with glycerol, indicating that glycerol, and not glycogen, is used directly as a carbon source under these mixotrophic conditions. Interestingly,hoxHexpression was also significantly downregulated in the presence of glycerol. Expression ofhupSwas lower under light. The presence ofcoxAtranscripts suggested respiratory activities in the vials under all conditions. 16SrRNAwas used as the loading control. –RTase denotes controls to demonstrate absence of DNA contamination in the samples. (c) Addition of NaNO3to the medium of an N2-fixing culture resulted in cessation of H2production (blue) within 12 h and greatly reduced nitrogen fixation (green). Nitrogenase activity is expressed in terms of ethylene production by acetylene reduction. Each column represents an average of measurements from at least three biological replicates. Error bars indicate s.d. values from the average. Full size image Figure 4: H 2 production in Cyanothece 51142 is primarily mediated by the nitrogenase enzyme system. ( a ) Comparisons of the expression of genes involved in H 2 metabolism under N 2 -fixing (−NO 3 ) and nitrogen-sufficient (+NO 3 ) conditions from cultures grown under 12 h light/dark cycles. nifH transcripts could only be observed under N 2 -fixing condition, whereas hoxH and hupS transcripts were present under both conditions. coxA transcripts were predominant during the dark cycle both under N 2 -sufficient and N 2 -deficient conditions. Transcripts for glgP were abundant during the dark cycle under both conditions. 16S rRNA was used as the loading control. Cells were collected at 4 h intervals, between D1 (1 h after the onset of the dark cycle) and L9 (9 h into the light cycle). ( b ) Reverse transcription PCR analysis of the enzyme systems involved in H 2 metabolism in Cyanothece 51142. Samples were collected from the incubation bottles (continuous light, aerobic) at the beginning (I 0 ) and end of the incubation phase (I 12 ). Strong nifH expression could be observed at I 0 , in the control (grown in ambient CO 2 ) as well as in cultures supplemented with high concentrations of CO 2 or glycerol. nifH transcripts were also present in cells incubated under light during H 2 production (I 12 ). Expression of glgP was downregulated in cultures supplemented with glycerol, indicating that glycerol, and not glycogen, is used directly as a carbon source under these mixotrophic conditions. Interestingly, hoxH expression was also significantly downregulated in the presence of glycerol. Expression of hupS was lower under light. The presence of coxA transcripts suggested respiratory activities in the vials under all conditions. 16S rRNA was used as the loading control. –RTase denotes controls to demonstrate absence of DNA contamination in the samples. ( c ) Addition of NaNO 3 to the medium of an N 2 -fixing culture resulted in cessation of H 2 production (blue) within 12 h and greatly reduced nitrogen fixation (green). Nitrogenase activity is expressed in terms of ethylene production by acetylene reduction. Each column represents an average of measurements from at least three biological replicates. Error bars indicate s.d. values from the average. Full size image Hydrogen production is mediated by the nitrogenase enzyme Genome analysis of Cyanothece 51142 revealed the presence of both the nitrogenase (Nif) and bidirectional hydrogenase (Hox) enzyme systems. Analysis at the transcriptional level revealed that hox genes were expressed under both nitrogen-fixing (−NO 3 ) and nitrogen-sufficient (+NO 3 ) conditions ( Fig. 4a ), and higher transcript abundance could be associated with the dark period under both conditions. In contrast, nif genes were expressed only under nitrogen-fixing conditions, and, in the absence of any additional carbon source, the nif transcripts were strictly associated with the dark period ( Fig. 4a ). High levels of H 2 production in Cyanothece 51142 were detected exclusively under diazotrophic conditions, and addition of combined nitrogen to the growth media of nitrogen-fixing cultures resulted in an immediate reduction in the rates of nitrogen fixation and simultaneous cessation of H 2 production ( Fig. 4c ). These results show that the high rates of H 2 production observed in Cyanothece 51142 were primarily mediated by the nitrogenase enzyme system. Nitrogenase can be optimized to enhance hydrogen yield An important feature of the nitrogenase enzyme system is the potential to channel all available electrons towards H 2 production in the absence of molecular nitrogen [26] , [27] . The nitrogenase reaction is also resistant to feedback inhibition from accumulated H 2 (ref. 28 ). When Cyanothece 51142 cells grown under photoautotrophic conditions were incubated under an argon atmosphere (absence of molecular nitrogen), a 2- to 3-fold increase (>370 μmol of H 2 per mg of Chl.h or 5.738 μmol of H 2 per mg of dry weight per hour) in the yield of H 2 was achieved ( Fig. 5 , Tables 1 and 2 ). In addition, production rates of up to 467 μmol of H 2 per mg of Chl.h were achieved from cells grown in glycerol-supplemented media subsequently incubated under argon environment ( Fig. 5 ). These rates are at least an order of magnitude higher compared with any other hydrogen-producing photosynthetic microbial wild-type strain studied to date ( Tables 1 and 2 ). 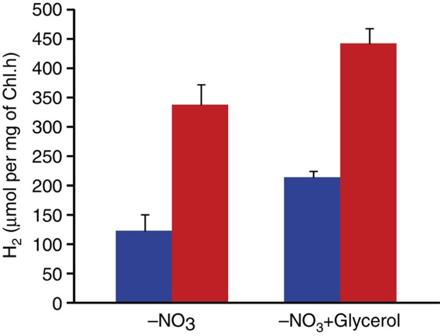Figure 5: Effect of argon environment on H2production inCyanothece51142. Higher specific rates of H2production are achieved in the absence of molecular N2in the headspace of the incubation bottles. Each column represents an average of measurements from at least three biological replicates in air (blue) and argon (red) atmospheres. Error bars indicate s.d. values from the average. Figure 5: Effect of argon environment on H 2 production in Cyanothece 51142. Higher specific rates of H 2 production are achieved in the absence of molecular N 2 in the headspace of the incubation bottles. Each column represents an average of measurements from at least three biological replicates in air (blue) and argon (red) atmospheres. Error bars indicate s.d. values from the average. Full size image Table 2 Full size table This work describes the use of the wild-type strain of the unicellular cyanobacterium Cyanothece 51142 for highly efficient photobiological H 2 production under natural aerobic conditions. In general, the oxygen sensitivity of the enzymes involved in biological H 2 production makes the use of oxygenic photosynthetic organisms as a platform for H 2 production an extremely challenging task. Thus, until now, photobiological H 2 production studies have largely relied on artificial interventions, which help to create an anaerobic environment. It has been recognized that the use of oxygenic photosynthetic microbes that can produce H 2 under aerobic conditions would be an important step forward for biological H 2 production [29] . Our study has identified Cyanothece 51142 as one such organism that has developed an effective strategy to make the best use of a diurnal cycle—synthesizing energy-rich storage compounds during the day and using it for nitrogen fixation at night when oxygen-consuming processes render the interior of the cell anaerobic (or suboxic), while the extracellular environment continues to be oxygen rich. This trait of Cyanothece 51142 formed the basis for the physiological perturbations that were designed for our two-stage aerobic H 2 production process. Nitrogen fixation is an energy-intensive process, requiring 16 molecules of ATP for every molecule of nitrogen fixed and H 2 produced [19] ( Fig. 1 ). However, the process is of paramount importance to diazotrophic species inhabiting ecological niches (such as deep oceans) with very low levels of nitrogenous nutrients. Consequently, photoautotrophic unicellular strains such as Cyanothece 51142 are expected to have evolved effective strategies for collecting and storing solar energy, which can be used at night when the energy demands are high. Our study shows that Cyanothece 51142 not only develops an intracellular environment conducive for the function of the nitrogenase enzyme but also generates an adequate supply of ATP for this high-energy-requiring process. In addition, our results reveal high specific activity of the nitrogenase enzyme in this strain, a finding consistent with earlier reports that showed higher rates of nitrogen fixation in marine unicellular diazotrophs such as Cyanothece compared with some filamentous strains [16] , [30] . A unicellular, marine, diazotrophic Synechococcus strain ( Synechococcus Miami BG 43511; later classified as Cyanothece Miami BG 43511 [16] ) was also shown to exhibit high rates of nitrogenase activity and hydrogen production [31] . Unfortunately, this strain has not been readily accessible to the general research community. Notably, not all unicellular cyanobacterial strains are endowed with these traits, as is evident from studies on Gloeothece , a unicellular freshwater diazotroph that possesses a nitrogenase enzyme with relatively low specific activity and does not have any appreciable nitrogenase-mediated H 2 production capacity [32] . Diazotrophic cyanobacteria have developed various strategies to protect their nitrogenase enzyme from the oxygen-rich environment they inhabit. However, unlike Cyanothece 51142, most diazotrophic strains are unable to exhibit nitrogenase-mediated H 2 production under aerobic conditions. In filamentous, heterocyst-forming diazotrophic strains, this is largely ascribed to the activities of an uptake hydrogenase enzyme system that is functionally closely associated with nitrogenase and oxidizes the H 2 produced [3] , [33] , [34] , [35] . It has been shown that wild-type Anabaena variabilis cells can generate H 2 only under an argon atmosphere, whereas its uptake hydrogenase mutants PK84 and AVM13 can produce H 2 aerobically [27] , [36] , [37] , [38] . A recent study also demonstrated H 2 production ( ∼ 25 μmol per mg of Chl.h) from the vegetative cells of wild-type Anabaena variabilis under nitrogen atmosphere when strict anaerobic conditions are maintained [39] . The genome sequence of Cyanothece 51142 shows the presence of hup genes for an uptake hydrogenase. The transcripts for one of these genes, hupS , were also detected under H 2 -producing conditions ( Fig. 4b ). Interestingly, the hupS transcripts in Cyanothece 51142 were present under both nitrogen-sufficient and nitrogen-fixing conditions ( Fig. 4a ), indicating that its expression is independent of nif . The presence of hupS transcripts and the concurrent accumulation of H 2 at high rates under aerobic incubation conditions are suggestive of a weak uptake hydrogenase activity in Cyanothece 51142. Such a premise is also supported by the observation that a few wild-type Anabaena strains that possess uptake hydrogenases with very low specific activities can also exhibit aerobic H 2 production [24] , [40] , [41] . The ability to use high concentrations of CO 2 or glycerol for enhanced H 2 production is an added advantage, as both of these carbon sources are abundantly available as industrial waste products, making biohydrogen production by Cyanothece 51142 an attractive option. High CO 2 and glycerol provide an additional carbon source and the availability of excess carbon functions as a signal for enhanced nitrogenase activity to meet the increase in nitrogen demand in these cyanobacterial cells. The rise in the glycogen level of cells at the end of the incubation phase in glycerol-supplemented cultures could be a result of cellular activities geared towards building energy reservoirs when an external energy source is readily available [21] . Decades of research have unveiled various principles underlying biological H 2 production. However, achieving significant increases in yield has been a major challenge. Genetic modifications of H 2 -yielding pathways have resulted in improvements in production rates compared with the corresponding wild-type strains [9] , [42] , [43] . However, as the H 2 production rates in these wild-type strains are rather modest, even a 20-fold increase in yield in mutant strains is not sufficient to attain a high production level. Therefore, our identification of a cyanobacterial strain exhibiting high rates of H 2 production under ambient aerobic conditions offers new possibilities in photobiological hydrogen production research. Recent studies have revealed the metabolic flexibility of this cyanobacterium [25] , and demonstrated that its robust circadian rhythm allows N 2 fixation and H 2 production to occur at reasonably high rates even when grown under continuous light [44] . Previous studies have shown the robustness of other cyanobacterial systems for H 2 production over a prolonged period of time [38] , demonstrating the possibility of using high-H 2 -yielding cyanobacterial strains for large-scale production. A systems level understanding of this biological phenomenon in Cyanothece 51142 will unravel previously unknown cellular factors and regulatory mechanisms that influence the process so that they can be favourably altered to produce even higher levels of H 2 as an energy carrier. Growth conditions For H 2 measurement, Cyanothece 51142 cells were grown in shaking flasks in ASP2 medium [45] without supplemented NaNO 3 at 30 °C under 12 h light/12 h dark cycles and 100 μmol photons per m 2 s −1 of white light. Cultures were inoculated with 0.25 volumes of cultures grown in ASP2 medium without NaNO 3 under continuous light (50 μmol photon per m 2 s −1 white light), which in turn were inoculated with 0.1 volumes of cultures grown in ASP2 with NaNO 3 under similar conditions. For photomixotrophic growth, cultures were supplemented with 50 mM glycerol. For growth under high-CO 2 conditions, the cultures were aerated with 8% CO 2 -enriched air at a flow rate of 100 ml min −1 . H 2 production and nitrogenase activity measurement A volume of 20 ml of culture was transferred at the beginning of the dark period to air-tight glass vials (36 ml) and incubated in air under a light intensity of 100 μmol photon per m 2 s −1 for 12 h. The chlorophyll content of cultures grown without an external carbon source ranged between 0.5 and 2 μg ml −1 , whereas cultures supplemented with glycerol had higher chlorophyll concentration (2–5 μg ml −1 ). Dry weight of photoautotrophically grown culture ranged between 90 and 98 μg ml −1 . For anaerobic incubation, the glass vials were flushed with argon for 15–30 min. For the batch culture experiment, 25 ml of dense (8–12 μg chlorophyll per ml culture) glycerol-supplemented culture was incubated in 145 ml vials under constant illumination. H 2 that accumulated in the headspace of sealed culture vials was withdrawn with an air-tight syringe and quantified using an Agilent 6890N Gas Chromatograph (Agilent) equipped with a Molsieve 5A 60/80 column (Molsieve; inner dimensions 6′×1/8″) and a thermal conductivity detector. Injection port, oven and detector temperatures were 100, 50 and 100 °C, respectively. Argon, the carrier gas, was supplied at a flow rate of 65 ml min −1 . The volume of gas expressed in the results section was under standard conditions (assuming 1 ml H 2 =44.6 μmol). Nitrogenase activity of the H 2 -producing cultures was determined using an acetylene reduction assay [46] and expressed in terms of the ethylene produced. Cells were incubated in sealed glass vials in light at 30 °C under a 5% acetylene atmosphere with or without flushing with argon. Gas samples were withdrawn, and ethylene production was measured using an Agilent 6890N Gas Chromatograph (Agilent) equipped with a Poropak N column (inner dimensions 5′×I/8″) and a flame ionization detector using argon as the carrier gas (flow rate of 65 ml min −1 ), according to the manufacturer's instructions. The temperature of the injector, detector and oven were 150, 200 and 100 °C, respectively. Total chlorophyll a was extracted by methanol and quantified spectrophotometrically using an Olis DW2000 spectrophotometer (On-Line Instrument Systems). Protein concentrations were determined using a bicinchoninic acid assay (Pierce) according to the manufacturer's instructions. Oxygen measurements O 2 concentrations in the headspace of the incubation vials were determined using an Agilent 6890N Gas Chromatograph (Agilent) equipped with a Molsieve 5A 60/80 column (Molsieve; inner dimensions 6′×1/8″) and a thermal conductivity detector using the same settings as described above for the H 2 assay. The measurements were taken under standard conditions. Dissolved O 2 concentration in the incubation vials was measured using a Clark-type electrode. Calculations were based on the fact that air-saturated water contains 230 μM of O 2 at 30 °C. Determination of glycogen content Samples were collected for the glycogen assay at the beginning and end of the 12 h-light incubation phase of H 2 production. The cellular glycogen content was measured using a glucose hexokinase assay (Sigma) with glycogen from bovine liver Type IX (Sigma) as standard. After methanol extraction of chlorophyll, the cell pellets were washed twice with 100% ethanol. To remove free glucose, 40% KOH was added and the samples were incubated for 1 h at 95 °C. Glycogen was precipitated overnight at −20 °C with 2 volumes of 100% ethanol. The samples were centrifuged for 1 h at 4 °C and 2 N HCl was added before incubation at 95 °C for 30 min. The same volume of 2 N NaOH and 0.5 volumes of 1 M phosphate buffer, pH 7, were added before dilution with 1 volume of distilled water. For the enzyme assay, 75 μl of sample solution was mixed with 200 μl of enzyme solution in a microtitre plate (Costar, ultraviolet light proof). After 15 min incubation at ambient temperature, NADPH was measured at 340 nm on a μQuant plate reader (Bio-Tek Instruments). Semiquantitative reverse transcription (RT–PCR) Semiquantitative RT–PCR analyses were performed on RNA samples isolated from cultures grown under nitrogen-fixing (−NO 3 ) conditions, with and without supplemented glycerol; from cultures grown under aeration with 8% CO 2 -enriched air; and under non-nitrogen-fixing conditions (+NO 3 ). For the time-course experiment, samples were collected every 4 h for 24 h, starting with 1 h into the dark period (D1). In total, six samples were collected. For RT–PCR analysis under H 2 -producing conditions, culture samples were assayed at the end of the light period at time point I 0 and from the assay bottles at the end of incubation at time point I 12 . RNA was isolated and quantified essentially as described in ref. 14 . A volume of 700 ng of DNase (Promega)-treated total RNA samples was used for reverse transcription with the Superscript II Reverse Transcriptase and random primers (Invitrogen) according to the manufacturer's instructions. The absence of DNA contamination was tested for each RNA sample ( Fig. 4b ). PCR was carried out at 94 °C for 4 min, followed by 94 °C for 30 s, 58 °C for 20 s, 72 °C for 20 s and a final extension time of 4 min at 72 °C. A total of 25 cycles for the nifH , hupS , glgP and coxA genes and 26 cycles for the hoxH gene were used. The following primers were used: nifH F: 5′-ACCATTGCTGCGTTAGCTGAAAC-3′, R: 5′-TAATACCACGACCCGCACATCCA-3′; coxA F: 5′-TGATATGGCCTTTCCCACCCTCA-3′, R: 5′-AGAGAACTAAAGCGGCAGCGAGA-3′; hupS F: 5′-ATAGCTGGTTTCGTTGTCGCTGT-3′, R: 5′-CGAAGTCTTGGGTGGTTGCTTTG-3′; hoxH F: 5′-TGGAGAAGACGGACTTTGGGAAC-3′, R: 5′-AAAGAAGAGGTCGCTACACCACC-3′; glgP F: 5′-TCGGCTGAATTCCTTATGGGTCG-3′, R: 5′-CAGGAATTTCCACTTGCCAACCG-3′; 16S rRNA F: 5′-AGAGGATGAGCAGCCACACT-3′, R: 5′-TAATTCCGGATAACGCTTGC-3′ (F: forward, R: reverse). How to cite this article: Bandyopadhyay, A. et al . High rates of photobiological H 2 production by a cyanobacterium under aerobic conditions. Nat. Commun. 1:139 doi: 10.1038/ncomms1139 (2010).